Atomically synergistic Zn-Cr catalyst for iso-stoichiometric co-conversion of ethane and CO2to ethylene and CO Developing atomically synergistic bifunctional catalysts relies on the creation of colocalized active atoms to facilitate distinct elementary steps in catalytic cycles. Herein, we show that the atomically-synergistic binuclear-site catalyst (ABC) consisting of \({{{{{\rm{Zn}}}}}}^{\delta+}\) -O-Cr 6+ on zeolite SSZ-13 displays unique catalytic properties for iso-stoichiometric co-conversion of ethane and CO 2 . Ethylene selectivity and utilization of converted CO 2 can reach 100 % and 99.0% under 500  °C at ethane conversion of 9.6%, respectively. In-situ/ex-situ spectroscopic studies and DFT calculations reveal atomic synergies between acidic Zn and redox Cr sites. \({{{{{\rm{Zn}}}}}}^{\delta+}\) ( \(0 \, < \, \delta \, < \, 2\) ) sites facilitate β-C-H bond cleavage in ethane and the formation of Zn-H δ - hydride, thereby the enhanced basicity promotes CO 2 adsorption/activation and prevents ethane C-C bond scission. The redox Cr site accelerates CO 2 dissociation by replenishing lattice oxygen and facilitates H 2 O formation/desorption. This study presents the advantages of the ABC concept, paving the way for the rational design of novel advanced catalysts. The synergistic effects generated by mixed or supported bifunctional catalysts are often claimed to promote the catalytic performance of traditional heterogeneous catalysts [1] , [2] , [3] , [4] , [5] , [6] , [7] , [8] , [9] . Recently, the construction of synergistic pair-sites with colocalized metal atoms to facilitate distinct elementary steps in the catalytic reaction has been established as a crucial step toward atomically synergistic bifunctional catalyst development [10] , [11] , [12] . The interaction between these adjacent metal atoms, similar to the metal-support interaction of traditional heterogeneous catalysts [3] , [13] , offers the possibility to modulate their respective electronic structure to further enhance their catalytic activity [11] , [14] , [15] , [16] , [17] . However, precisely controlling their colocalization requires a complicated synthesis process with multiple synthesis steps to load single atoms [10] , [18] . Moreover, the stability of the well-defined synergistic sites is debatable, especially under harsh reaction conditions such as high reaction temperatures [18] , [19] . The benefits and remaining challenges of atomically synergistic bifunctional catalysts motivate us to further explore new synthesis routes, new reaction applications, and their synergistic effects with the goals to accelerate the development of next-generation atomically synergistic catalysts. Growing CO 2 emissions and abundant shale gas reserves have prompted a significant amount of research to explore efficient approaches for co-utilizing the products to produce value-added chemicals [20] , [21] , [22] . Ethane, the second-largest component of shale gas, is an ideal alternative hydrogen source for CO 2 conversion. The co-conversion of ethane and CO 2 (C 2 H 6 + CO 2 → C 2 H 4 + CO + H 2 O) is a viable alternative to the ethane steam cracking for ethylene production under the goal of net negative CO 2 emissions [21] . Furthermore, iso-stoichiometric co-conversion of ethane and CO 2 (ICEC) to ethylene and CO is crucial for direct downstream processes such as the hydroformylation reaction to produce aldehyde [23] and polymerization process to produce polyketones [24] , [25] , [26] , [27] . However, the ICEC process lacks a viable catalyst for achieving high ethylene selectivity and CO 2 utilization simultaneously. Metal-based catalysts suffer from the inevitable cleavage of C-C bonds through dry reforming pathways and lower the ethylene selectivity [22] , [28] , [29] , [30] . Oxide-based catalysts exhibit the great merit of preferential C–H bond scission over C–C bond scission pathways but require excessive CO 2 cofeeding to reduce ethane adsorption and scavenge the surface H species [31] , [32] . Specifically, Zn and Cr oxide-based catalysts were widely studied for co-conversion of ethane and CO 2 . The acidic Zn 2+ site displayed high activity for C-H bond cleavage in ethane and CO 2 activation, requiring the participation of adjacent active sites to form binuclear sites [33] , [34] , [35] . The challenge is that acidified Zn 2+ -H hydride displays a capacity for C-C bond scission of ethane, leading to undesired production of methane. Redox Cr 6+ sites require lattice oxygen as a H acceptor to dissociate C-H bonds but trigger the formation of less active Cr 3+ species. The reoxidation of Cr 3+ to Cr 6+ is limited by slow O abstraction from CO 2 [20] . The above analyses thus indicate the need for the development of an atomically-synergistic binuclear Zn–O–Cr site catalyst for ICEC, with Zn facilitating CO 2 adsorption and activation to provide O species for Cr 6+ regeneration and adjacent Cr as an electron donor reducing the acidity of Zn 2+ to facilitate its activity and selectivity for C-H bond scission [6] , [36] , [37] , [38] , [39] . More generally, exploring a cooperative redox and acid-base catalytic mechanism for ICEC is highly desirable. In this work, we show the successful fabrication and demonstration of a Zn-O-Cr atomically-synergistic binuclear-site catalyst (ABC) that is highly efficient for ICEC with high ethylene selectivity and utilization of converted CO 2 ( \({{{{{\rm{U}}}}}}_{{{{{{\rm{CO}}}}}}_{2}}\) ). As we will show, compared with pure Zn and Cr catalysts, Zn-O-Cr ABC displays ~1.5 and ~4-fold higher catalytic activity with 100% ethylene selectivity and 99.0% \({{{{{\rm{U}}}}}}_{{{{{{\rm{CO}}}}}}_{2}}\) under optimized reaction conditions. Key to this high performance is the discovery that Cr facilitates the formation of a \({{{{{\rm{Zn}}}}}}^{\delta+}\) ( \(0 \, < \, \delta \, < \, 2\) ) site to enhance the β-C-H bond cleavage of ethane, while the resulting Lewis base Zn-H δ - hydride favors CO 2 adsorption and activation, and prevents C-C bond scission of ethane. The redox Cr site accelerates CO 2 dissociation and facilitates H 2 O formation/desorption. The apparent activation energies of ethane conversion and CO 2 conversion are ~70.9 and ~74.0 kJ/mol, which demonstrates the rate matching achieved in ICEC. Controlling Zn and Cr coordination structure Catalysts were synthesized by mixing a constant total amount of zinc (II) acetate and chromium (III) acetate hydroxide on a SSZ-13 zeolite support with varying Zn/Cr molar ratios, followed by direct decomposition at 550°C and then Na + neutralization of acidic site on supports (Fig. 1a ). The catalyst synthesis method developed here will be referred to as the dry-deposition method (The experimental details are summarized in Methods). The catalysts are denoted as Zn x Cr y /SSZ-13, where x/y refers to the ratio of Zn/Cr ( x = 1, y = 0; x/y = 1/2, 1, 2, 3, 4; x = 0, y = 1). The textural properties, composition analysis, and surface acidity of SSZ-13 and synthesized catalysts are characterized by N 2 physisorption, X-ray fluorescence (XRF), and attenuated total reflection Fourier transform infrared (ATR-FTIR) measurements (Supplementary Figs. 1 - 2 and Tables 1 - 2 ). Transmission electron microscopy (TEM), scanning TEM (STEM) images, and energy dispersive spectroscopy (EDS) elemental mappings (Fig. 1b and Supplementary Figs. 3 - 5 ) demonstrate high dispersion of Zn and/or Cr oxide phases, with no observable sintering of oxide nanoparticles. The X-ray diffraction (XRD) results reveal the absence of spinel ZnCr 2 O 4 and zincite ZnO for all dry-deposition synthesized catalysts. Cr 2 O 3 phases with R3c space group were only observed in Cr/SSZ-13 and Zn 1 Cr 2 /SSZ-13 (Supplementary Fig. 6 ). The control samples with same amount Zn and Cr precursors were prepared via a co-precipitation method (CP), followed by Na + neutralization. ZnCrO x nanoparticles are observed in CP-synthesized samples (Supplementary Fig. 7 ). And a phase transition from spinel ZnCr 2 O 4 to ZnO (Supplementary Fig. 8 ) was detected on CP-synthesized catalysts with Zn/Cr ratios varying from 1/2 to 3/1 [40] , [41] , [42] . Fig. 1: Coordination of Zn-O-Cr sites in atomically-synergistic binuclear-site catalyst (ABC). a Schematic illustration of the fabrication process of Zn-O-Cr ABC. b Representative TEM and HAADF-STEM images and EDS mapping of Zn-O-Cr ABC with Zn/Cr ration of 3/1; c The proportion of Zn δ + \((0 \, < \, \delta \, < \, 2)\) (left) and Cr 6+ (right) with varying Zn/Cr ratios (Results derived from Auger spectra of Zn LMM and Cr 2 p 3/2 XPS spectra); d Enlarged electron transition features in Zn and Cr K-edge XANES spectra; e k 3 -weighted Fourier-transformed extended X-ray absorption fine structure (FT-EXAFS) spectra (Zn K-edge ) of Zn-O-Cr ABCs with varying Zn/Cr ratios, with Zn foil and ZnO as references; f Coordination number (CN) of Zn-O-Cr(Zn) and Cr-O in Cr 6+ state in Zn-O-Cr ABCs with varying Zn/Cr ratios. 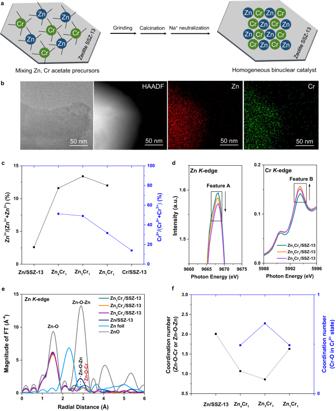Fig. 1: Coordination of Zn-O-Cr sites in atomically-synergistic binuclear-site catalyst (ABC). aSchematic illustration of the fabrication process of Zn-O-Cr ABC.bRepresentative TEM and HAADF-STEM images and EDS mapping of Zn-O-Cr ABC with Zn/Cr ration of 3/1;cThe proportion of Znδ+\((0 \, < \, \delta \, < \, 2)\)(left) and Cr6+(right) with varying Zn/Cr ratios (Results derived from Auger spectra of ZnLMMand Cr 2p3/2XPS spectra);dEnlarged electron transition features in Zn and CrK-edgeXANES spectra;ek3-weighted Fourier-transformed extended X-ray absorption fine structure (FT-EXAFS) spectra (ZnK-edge) of Zn-O-Cr ABCs with varying Zn/Cr ratios, with Zn foil and ZnO as references;fCoordination number (CN) of Zn-O-Cr(Zn) and Cr-O in Cr6+state in Zn-O-Cr ABCs with varying Zn/Cr ratios. Full size image Figure 1c , Supplementary Figs. 9 - 11 and Supplementary Table 3 show X-ray photoelectron spectroscopy (XPS) results for Zn 2 p , Zn LMM Auger and Cr 2 p 3/2 spectra. 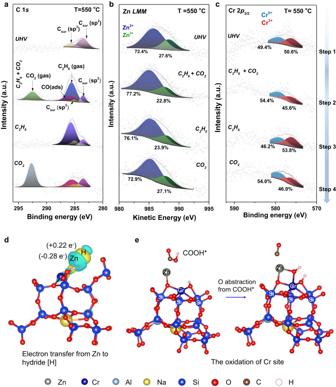Fig. 3: Electronic structure changes of binuclear Znδ+-O-Cr6+sites. In situ ambient pressure X-ray photoelectron spectroscopy (APXPS):aC 1sspectra,bAuger spectra of ZnLMM, andcCr 2p3/2spectra as a function of reaction conditions for Zn3Cr1/SSZ-13. T = 550  °C: ultra-high vacuum (UHV), C2H6(50 mTorr) + CO2(50 mTorr), C2H6(100 mTorr), and CO2(100 mTorr) in sequence.dElectron transfer from Zn to H after the 2ndC-H bond scission in ethane (H: white; Zn: gray), where electron accumulation and depletion are represented by yellow (Δρ = +1 × 10−3e bohr−3) and cyan (Δρ = −1 × 10−3e bohr−3) respectively.eThe oxidation of Cr in Zn-O-Cr when decomposing COOH* intermediate. The formation of Zn δ + (0 < δ < 2) was confirmed through Auger spectra of Zn LMM . The subpeaks at 987.5 and 990.0 eV in Auger spectra of Zn LMM (Supplementary Fig. 10 ) are assigned to the Zn 2+ and \({{{{{\rm{Zn}}}}}}^{\delta+}\) ( \(0 \, < \, \delta \, < \, 2\) ), respectively; [43] And the subpeaks at ~576 and ~580 eV in Cr 2 p 3/2 XPS (Supplementary Fig. 11 ) were assigned to the Cr 3+ and Cr 6+ , correspondingly [44] . Figure 1c shows the proportion of \({{{{{\rm{Zn}}}}}}^{\delta+}\) 0 < δ < 2 and Cr 6+ relative to the total amount of \(({{{{{\rm{Zn}}}}}}^{\delta+}+{{{{{\rm{Zn}}}}}}^{2+})\) and (Cr 6+ +Cr 3+ ) in Zn x Cr y /SSZ-13 catalysts, respectively. These proportions vary with Zn/Cr ratios, with the highest Zn δ + (0 < δ < 2) proportion generated at Zn/Cr ratio of 3/1 and the highest Cr 6+ proportions produced at Zn/Cr ratios of 3/1 and 4/1. We hypothesize that the proximal electronic interactions between Zn and Cr could modify their respective oxidation states. This is consistent with the Zn L 3 -edge X-ray absorption near-edge structure (XANES) spectra analyses (Supplementary Fig. 12 ), which suggests a decrease in the oxidation state of Zn in Zn x Cr y /SSZ-13 samples compared to pure Zn/SSZ-13 sample. The \({{{{{\mathrm{Zn}}}}}}^{\delta+}\) and Cr 6+ content in the CP-synthesized Zn 3 Cr 1 /SSZ-13 sample is similar to those of pure Zn/SSZ-13 and Cr-SSZ-13 samples, respectively (Supplementary Fig. 13 ). XANES spectra (Fig. 1d and Supplementary Fig. 14 ) and extended X-ray absorption fine structure (EXAFS) spectra (Fig. 1 e, f, Supplementary Figs. 15 – 18 , Supplementary Tables 4 - 5 ) were used to study coordination structures of Zn and Cr sites. As shown in Fig. 1d and Supplementary Fig. 14 , the electron transition from Zn 1 s to Zn 4 p unoccupied orbitals (Feature A) is revealed in Zn K -edge XANES spectra; and Cr K -edge XANES spectra exhibits the peak of electron transition from Cr 1 s to Cr 3 d -O 2 p unoccupied orbitals (Feature B). As the Zn/Cr ratio increases from 1/1 to 4/1 in Zn x Cr y /SSZ-13 catalysts, the intensity of feature A decreases, suggesting electron occupation in Zn 4 p unoccupied orbitals, while the intensity of feature B increases, which suggests electrons transfer out of Cr 3 d -O 2 p orbitals near the conduction band minimum. We hypothesize a link between these observations, that electronic charge transfers from Cr 3 d -O 2 p character in the conduction band to Zn 4 p [45] , [46] , due to a strong Zn-Cr interaction. Thus, the charge transfer decreases the oxidative state of Zn 2+ to \({{{{{\rm{Zn}}}}}}^{\delta+}\) ( \(0 \, < \, \delta \, < \, 2\) ), which is consistent with XPS and Auger results (Fig. 1c ). In Fig. 1e , the scattering peaks at 1.50 Å are assigned to Zn-O coordination in the first shell. The pure Zn/SSZ-13 and Zn x Cr y /SSZ-13 samples exhibited a significantly lower intensity for this Zn-O scattering peak than the ZnO reference, suggesting a higher degree of crystal disorder [47] , [48] . The scattering peaks at ~2.85 Å are assigned to Zn-O-Zn coordination in the second shell. Compared to Zn/SSZ-13 and the ZnO reference, Zn 1 Cr 1 /SSZ-13 and Zn 3 Cr 1 /SSZ-13 exhibited no peak for Zn-O-Zn coordination. Instead, a new peak at ~3.08 Å should be attributed to the Zn-O-Cr bond [41] . Differently, Zn 4 Cr 1 /SSZ-13 sample has both Zn-O-Cr and Zn-O-Zn bonds. Cr K -edge Fourier transformed EXAFS (FT-EXAFS) spectra of Cr-containing samples (Supplementary Fig. 15 ) displayed Cr-O scattering peaks located at 1.51 Å, which is similar to standard peak of Cr-O scattering 1.50 Å in Cr III 2 O 3 ; but as Zn/Cr ratio increase to 3/1 and 4/1, a visible shoulder peak corresponding to standard peak of Cr-O scattering at 1.20 Å in K 2 Cr VI 2 O 7 appeared, indicating that Zn 3 Cr 1 /SSZ-13 and Zn 4 Cr 1 /SSZ-13 samples have two types of Cr-O coordination. Supplementary Tables 4 - 5 show the EXAFS-derived fitting parameters. Zn x Cr y /SSZ-13 catalyst ( x/y = 1, 3, 4) samples show Zn-O-Cr coordination with a bond distance ~3.4 Å in phase-corrected space, which corresponds to the emergent peak at ~3.08 Å in Fig. 1e [41] . These results provide solid evidence for the formation of a Zn δ + -O-Cr 6+ structure in Zn x Cr y /SSZ-13. Notice that Zn x Cr y /SSZ-13 samples also exhibited lower coordination numbers (CNs) for Zn-O and Zn-O-Cr compared to the pure Zn/SSZ-13 sample (Fig. 1f and Supplementary Table 4 ), which results from Cr colocalization. 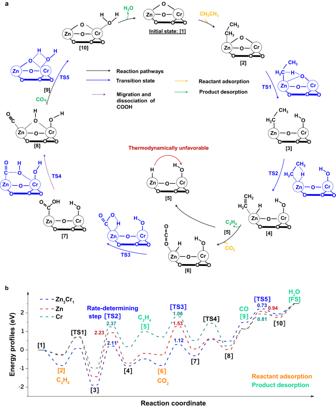Fig. 4: Atomically synergistic mechanism of ICEC over binuclear Zn-O-Cr sites. aCatalytic cycles of ICEC over binuclear Zn-O-Cr sites of Zn3Cr1/SSZ−13.bThe calculated energy profiles of ICEC on Zn3Cr1/SSZ−13, Zn/SSZ-13, and Cr/SSZ-13. Especially, for the Zn 3 Cr 1 /SSZ-13 and Zn 4 Cr 1 /SSZ-13 samples, the CNs of Zn-O and Zn-O-Cr are 3.94 and 0.86, and 3.77 and 1.07, respectively. 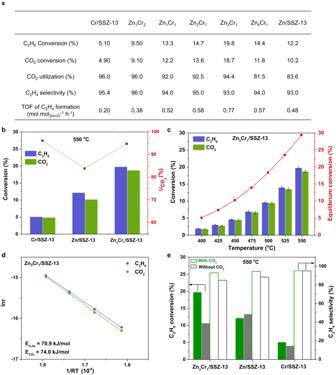And Zn 3 Cr 1 /SSZ-13 has the highest CN for the Cr-O bond in hexavalent (Cr 6+ ) states. Therefore, these results confirm the formation of hetero binuclear Zn δ + -O-Cr 6+ sites, and Zn 3 Cr 1 /SSZ-13 exhibits the highest population of the Zn δ + -O-Cr 6+ site. Fig. 2: Iso-stoichiometric co-conversion of ethane and CO2(ICEC). aCatalytic performance of Zn-O-Cr ABCs (Reaction condition: Temperature = 550  °C; Reactant composition = 5% C2H6+ 5% CO2+ 90% Ar; WHSV = 7500 mL g−1cath−1);bC2H6and CO2conversion, utilization of converted CO2(\({{{\mbox{U}}}}_{{{{{{\rm{CO}}}}}}_{2}}\)) of Cr/SSZ-13, Zn/SSZ-13, and Zn3Cr1/SSZ-13 catalysts in ICEC at 550  °C;cReaction temperature dependent performance of Zn3Cr1/SSZ-13 catalyst.dArrhenius plots of Zn3Cr1/SSZ-13 catalyst (obtained when both C2H6and CO2conversions are <10 %).eC2H6conversion and C2H4selectivity over Zn3Cr1/SSZ-13, Zn/SSZ-13, and Cr/SSZ-13 with (green columns) /without (gray columns) CO2at 550  °C. Catalytic performance of Zn-O-Cr ABC for ICEC Figure 2a, b and Supplementary Fig. 19 and Table 6 show the ICEC catalytic performance of Zn-O-Cr ABCs under the reaction conditions of weight hourly space velocity (WHSV) of 7500 mL g −1 cat h −1 and a CO 2 /ethane ratio of 1 at 550  °C. The Zn 3 Cr 1 /SSZ-13 ABC catalyst displayed the best performance among all tested catalysts, with the highest C 2 H 6 conversion (19.8%), CO 2 conversion (18.7%), turnover frequency (TOF) of C 2 H 4 formation (0.77 mol mol Zn+Cr −1 h −1 ), as well as excellent C 2 H 4 selectivity (93.0%) and \({{{{{\rm{U}}}}}}_{{{{{{\rm{CO}}}}}}_{2}}\) (94.4%). Previous studies have mainly focused on achieving high ethane conversion and ethylene selectivity in co-conversion of ethane and CO 2 by co-feeding excess CO 2 at CO 2 /ethane ratios of 2–6 [49] , [50] , [51] , [52] , [53] . In the ICEC process the C 2 H 4 selectivity and \({{{{{\rm{U}}}}}}_{{{{{{\rm{CO}}}}}}_{2}}\) are two important factors for evaluating the success of catalyst development. Utilization of converted CO 2 ( \({{{{{\rm{U}}}}}}_{{{{{{\rm{CO}}}}}}_{2}}\) ) is defined as the ratio of CO 2 conversion to ethane conversion on an iso-stoichiometric basis. Compared with previous studies in Supplementary Table 7 and Fig. 21 , the Zn 3 Cr 1 /SSZ-13 catalyst displays the highest space-time yield (STY) of C 2 H 4 formation (0.086 kg h −1 kg cat −1 ) and the highest \({{{{{\rm{U}}}}}}_{{{{{{\rm{CO}}}}}}_{2}}\) at 550 °C, which clearly shows the superiority of Zn–O–Cr ABCs. Furthermore, Fig. 2c and Supplementary Table 7 show C 2 H 4 selectivity can achieve 100% and \({{{{{\rm{U}}}}}}_{{{{{{\rm{CO}}}}}}_{2}}\) is 99.0% under the reaction temperature of 500  °C, with ethane conversion of 9.6% and CO 2 conversion of 9.5%. These results further demonstrate the advantage of Zn-O-Cr ABCs suitable for ICEC. In ICEC, the reaction system includes the reactants’ (ethane and CO 2 ) adsorption, activation, reaction, and products’ (ethylene, CO, and H 2 O) formation, and desorption. The apparent activation energies (E a ) for ethane conversion and CO 2 conversion are key to evaluating the rate matching of both reactions. Figure 2d shows similar E a (results were calculated based on Fig. 2c and Supplementary Fig. 22 ) for ethane dehydrogenation (70.9 kJ/mol) and CO 2 hydrogenation (74.0 kJ/mol). This further demonstrates the feasibility and success of the Zn-O-Cr ABCs concept for desired ICEC catalyst development. Fig. 2: Iso-stoichiometric co-conversion of ethane and CO 2 (ICEC). a Catalytic performance of Zn-O-Cr ABCs (Reaction condition: Temperature = 550  °C; Reactant composition = 5% C 2 H 6 + 5% CO 2 + 90% Ar; WHSV = 7500 mL g −1 cat h −1 ); b C 2 H 6 and CO 2 conversion, utilization of converted CO 2 ( \({{{\mbox{U}}}}_{{{{{{\rm{CO}}}}}}_{2}}\) ) of Cr/SSZ-13, Zn/SSZ-1 3 , and Zn 3 Cr 1 /SSZ-13 catalysts in ICEC at 550  °C; c Reaction temperature dependent performance of Zn 3 Cr 1 /SSZ-13 catalyst. d Arrhenius plots of Zn 3 Cr 1 /SSZ-13 catalyst (obtained when both C 2 H 6 and CO 2 conversions are <10 %). e C 2 H 6 conversion and C 2 H 4 selectivity over Zn 3 Cr 1 /SSZ-13, Zn/SSZ-13, and Cr/SSZ-13 with (green columns) /without (gray columns) CO 2 at 550  °C. Full size image Figure 2a and Supplementary Fig. 19 reveal that there is a clear correlation between the proportion of Zn δ + -O-Cr 6+ sites and ICEC performance. Pure Cr/SSZ-13 catalyst displayed slightly higher ethylene selectivity (95.4%) and higher \({{{{{\rm{U}}}}}}_{{{{{{\rm{CO}}}}}}_{2}}\) (96.0%) than Zn 3 Cr 1 /SSZ-13 sample, but has the lowest C 2 H 6 conversion (5.1 %), CO 2 conversion (4.9%), TOF of C 2 H 4 formation (0.20 mol mol Zn+Cr −1 h −1 ). Increasing Zn contents in Zn-O-Cr ABCs, with Zn/Cr ratios from 1/2 to 3/1, has little effect on ethylene selectivity and \({{{{{\rm{U}}}}}}_{{{{{{\rm{CO}}}}}}_{2}}\) . Instead, increased Zn contents promote higher conversion of C 2 H 6 and CO 2 , and leads to increased TOF of ethylene formation. Further increasing the Zn content to Zn/Cr ratio of 4/1, triggers lower ethane (14.4%) and CO 2 (11.7%) conversions, resulting in a much lower \({{{{{\rm{U}}}}}}_{{{{{{\rm{CO}}}}}}_{2}}\) (81.5 %). Pure Zn/SSZ-13 exhibited further decreased C 2 H 6 (12.1%) and CO 2 (10.2%) conversions, compared with Zn 4 Cr 1 /SSZ-13. Therefore, we hypothesize that the Zn δ + in the binuclear site of Zn δ + -O-Cr 6+ is the primary active site for C 2 H 6 dehydrogenation. Interestingly, the Zn δ + proportion also displays a correlation with CO 2 conversion, which indicates that the Zn δ + sites are also involved in CO 2 adsorption, activation, or reaction. In previous studies, binuclear Zn-O-Zn catalysts have been reported to have a high activity in ethane or propane dehydrogenation, but lack the capacity of efficient CO 2 activation, leading to insufficient CO 2 utilization [35] , [54] , [55] . In our study, the Zn 3 Cr 1 /SSZ-13 ABC with the highest amount of Zn δ + -O-Cr 6+ sites displayed ~1.5 and ~4-fold higher ethane dehydrogenation and CO 2 conversion performance than pure Zn and Cr catalysts, respectively (Fig. 2b ), which indicates the Cr 6+ site of Zn δ + -O-Cr 6+ is also involved in the activation and reaction of C 2 H 6 and CO 2 . From the above analyses, we conclude that the unique performance of Zn-O-Cr ABCs for ICEC relies on the atomic synergies within the Zn δ + -O-Cr 6+ site. To study the atomic synergies between Zn δ + -O-Cr 6+ site in ICEC, we compared the C 2 H 6 dehydrogenation performance of Zn 3 Cr 1 /SSZ-13 with pure Zn/SSZ-13 and Cr/SSZ−13 samples in the presence and absence of CO 2 . In Fig. 2e , we found the CO 2 co-feeding significantly improved C 2 H 6 conversion (19.8% vs. 10.7%) and C 2 H 4 selectivity (93.0% vs. 85.0%) for Zn 3 Cr 1 /SSZ-13, with a high \({{{{{\rm{U}}}}}}_{{{{{{\rm{CO}}}}}}_{2}}\) up to 94.4%. By contrast, for Zn/SSZ−13, CO 2 addition fails to enhance its C 2 H 6 conversion (12.1% vs. 13.3%) but results in an increase in C 2 H 4 selectivity (94.6% vs. 86.0%). The higher C 2 H 4 selectivity is due to competitive adsorption of CO 2 over C 2 H 6 , preventing the ethane cracking reaction, which has been reported previously [56] . Compared with Zn/SSZ−13, the improved C 2 H 6 conversion of the Zn 3 Cr 1 /SSZ-13 catalyst is due to the generation of Zn δ + in Zn δ + -O-Cr 6+ . For the Cr/SSZ−13 sample, CO 2 introduction results in a higher C 2 H 6 conversion (5.1% vs 4.0%) with a high \({{{{{\rm{U}}}}}}_{{{{{{\rm{CO}}}}}}_{2}}\) of 96%, but it did not change the C 2 H 4 selectivity (95.4% vs 95.1%). Cr-based catalysts are reported to catalyze CO 2 and ethane conversion through the redox (or MvK) mechanism [20] . CO 2 introduction could favor lattice oxygen replenishment to regenerate highly reactive Cr 6+ species and shift the reaction equilibrium of C 2 H 6 dehydrogenation, thus leading to a higher activity. These results indicate that a reaction synergy between ethane and CO 2 conversions could only occur at the atomically synergistic Zn δ + -O-Cr 6+ site. To further validate the superiority of Zn-O-Cr ABCs, we compared the performance of Zn 3 Cr 1 /SSZ−13 prepared by the dry-deposition method with the sample synthesized by the traditional co-precipitation (CP) method. Supplementary Fig. 23 shows that the dry-deposition synthesized Zn 3 Cr 1 /SSZ-13 catalyst exhibited >4-fold higher ethane conversion (19.8% vs 4.5%) and higher \({{{{{\rm{U}}}}}}_{{{{{{\rm{CO}}}}}}_{2}}\) (94.4% vs 83.2%). The CP-synthesized Zn 3 Cr 1 /SSZ-13 sample was found to contain large Zn/Cr oxide particles and separate ZnCr 2 O 4 and ZnO phases, resulting in loss of the atomic synergies of the Zn δ + -O-Cr 6+ site, which we correlate with its poor performance. We also studied the stability and regeneration ability of the Zn 3 Cr 1 /SSZ-13 ABC catalyst. Supplementary Fig. 24 shows that the ethylene selectivity and \({{{{{\rm{U}}}}}}_{{{{{{\rm{CO}}}}}}_{2}}\) remained nearly 100% during a total of 150 h in 3 cycles. And the decayed conversion of ethane and CO 2 can be totally regenerated by oxidative treatment in air at 500 °C. This excellent durability and regeneration ability demonstrates the structural stability of Zn δ + -O-Cr 6+ site. Electronic structure of binuclear Zn δ + -O-Cr 6+ sites during the reaction In situ ambient pressure X-ray photoelectron spectroscopy (APXPS) was employed to examine the electronic structure of binuclear Zn δ + -O-Cr 6+ sites and study the atomic synergies between Zn δ + and Cr 6+ sites in ICEC. Figure 3 a–c shows ambient pressure spectra indicating C 1 s binding energies, Zn LMM Auger kinetic energies, and Cr 2 p 3/2 binding energies. Fig. 3: Electronic structure changes of binuclear Zn δ + -O-Cr 6+ sites. In situ ambient pressure X-ray photoelectron spectroscopy (APXPS): a C 1 s spectra, b Auger spectra of Zn LMM , and c Cr 2 p 3/2 spectra as a function of reaction conditions for Zn 3 Cr 1 /SSZ-13. T = 550  °C: ultra-high vacuum (UHV), C 2 H 6 (50 mTorr) + CO 2 (50 mTorr), C 2 H 6 (100 mTorr), and CO 2 (100 mTorr) in sequence. d Electron transfer from Zn to H after the 2 nd C-H bond scission in ethane (H: white; Zn: gray), where electron accumulation and depletion are represented by yellow (Δρ = +1 × 10 −3 e bohr −3 ) and cyan (Δρ = −1 × 10 −3 e bohr −3 ) respectively. e The oxidation of Cr in Zn-O-Cr when decomposing COOH* intermediate. Full size image Step 1: Zn 3 Cr 1 /SSZ-13 was first tested under 550 °C in an ultra-high vacuum (UHV). The temperature of 550 °C was used to match the reaction temperature in Fig. 2 . In Auger spectra of Zn LMM (Fig. 3b ), both Zn 2+ (dark blue) and Zn δ + (green) species were detected with a percentage distribution of 72.4% and 27.6%, respectively. In Fig. 3c , Cr 3+ (dark red) and Cr 6+ (light blue) were detected with a proportion of 50.6% and 49.4%, respectively. Step 2: Then the Zn 3 Cr 1 /SSZ-13 was subjected to simulated reaction conditions of ICEC by co-feeding 50 mTorr C 2 H 6 and 50 mTorr CO 2 under 550 °C. The signals of gaseous C 2 H 6 and CO 2 were detected in Fig. 3a . Notably, adsorbed CO species (CO ads ) at 285.5 eV were observed [57] , [58] , which indicates the ICEC reaction occurred. Under the reaction conditions, the proportion of Zn δ + decreased (from 27.6% to 22.8%) and Cr 6+ ratio increased (from 49.4% to 54.4%). DFT calculations (Fig. 3d ) indicate that the oxidation from Zn δ + to Zn 2+ is due to the formation of Zn-H δ - hydride during the ethane dehydrogenation, with more negative charge accumulated on H δ - . The oxidation of Cr 3+ to Cr 6+ may result from lattice oxygen replenishment via CO 2 dissociation [20] . These results indicate both Zn δ + and Cr 6+ were involved in the ICEC reaction. Steps 3 and 4 were designed to understand the role of individual Zn δ + or Cr 6+ in ICEC. When feeding 100 mTorr C 2 H 6 (without CO 2 ) in step 3 (Fig. 3a, b ), the signals of CO 2 and CO ads species disappeared, which indicates that only ethane dehydrogenation could occur. The proportions of Zn 2+ and Zn δ + remain similar to the case of co-feeding C 2 H 6 and CO 2 in step 2, indicating the formation of Zn-H δ - hydride during the ethane dehydrogenation. Notice that the proportions of Zn δ + and Zn 2+ are comparable between step 1 (UHV) and step 4 (feeding 100 mTorr CO 2 without ethane), ruling out the likelihood of oxidation of Zn δ + to Zn 2+ by CO 2 or its derived intermediates. In the case of Cr 2 p 3/2 XPS spectra (Fig. 3c ), the oxidation of Cr 3+ to Cr 6+ only occurs when CO 2 was fed (steps 2 and 4). Previous studies have demonstrated the oxidation of Cr 3+ to Cr 6+ in Cr-based catalysts suffers from sluggish O abstraction from CO 2 [20] , [59] . In our cases, the facile reoxidation of Cr 3+ to Cr 6+ may be due to the possibility that nearby \({{{{{\rm{Zn}}}}}}^{\delta+}\) facilitate the CO 2 activation to enable easier O abstraction. The CO ads species at 285.5 eV were detected in the presence/co-presence of CO 2 in the C 1 s spectra (Fig. 3a , steps 2 and 4), which further demonstrates facile CO 2 dissociation over the Zn δ + -O-Cr 6+ site. Our DFT calculation (Fig. 3e ) indicates that the intermediate of CO 2 activation is carboxyl (COOH*). The decomposition of COOH* requires the participation of the Cr site through the formation of a new Cr-O bond (d(Cr-O) = 2.08 Å), which will maintain its high oxidation state. In summary, the APXPS results show that binuclear Zn δ + -O-Cr 6+ sites serve as atomically synergistic sites for ICEC. Atomically synergistic mechanism We developed atomically synergistic mechanisms for ICEC on binuclear Zn-O-Cr sites (Fig. 4 and Supplementary Fig. 30 - 35 , Supplementary Tables 8 - 10 ). Figure 4a shows that the catalytic cycle is initiated by C 2 H 6 adsorption on Zn ([1] [2]), then heterolytic cleavage of the first C-H bond (0.93 eV) by breaking a Zn-O-Cr bond to form Zn-CH 2 -CH 3 and Cr-OH ([2] [3]), followed by a homolytic scission of the β-C-H bond (2.11 eV) ([3] [4]), and finally, C 2 H 4 desorption and Zn-H δ - hydride formation ([4] [5]). C 2 H 6 activation at the Cr of Zn-O-Cr sites has higher energy barriers for the first C-H cleavage (1.78 eV vs 0.93 eV) and β-C-H bond dissociation (>3.0 eV vs 2.11 eV), leading to a kinetically unfavorable pathway (Supplementary Figs. 31 and 32 ). In the second stage (Fig. 4a ), CO 2 prefers to adsorb at Zn-H δ - site (−0.35 eV) than the Cr site (−0.05 eV) through acid-base interaction (Supplementary Fig. 33 ) ([5][6]) [60] , [61] ; CO 2 adsorption energy (−0.35 eV) at Zn-H δ - site is lower than ethane adsorption (−0.17 eV), which will help prevent the C 2 H 6 cracking reaction (Supplementary Table 5 ). Then Zn-H δ - enables CO 2 hydrogenation ([6][7]) to carboxyl (COOH*), followed by CO-OH cleavage and migration of -OH to be shared with Cr ([7][8]). Finally, after CO desorption from the Zn site and the formation and desorption of H 2 O from the Cr site to replenish lattice oxygen ([8][10]), the ICEC catalytic cycle is closed. Fig. 4: Atomically synergistic mechanism of ICEC over binuclear Zn-O-Cr sites. a Catalytic cycles of ICEC over binuclear Zn-O-Cr sites of Zn 3 Cr 1 /SSZ−13. b The calculated energy profiles of ICEC on Zn 3 Cr 1 /SSZ−13, Zn/SSZ-13, and Cr/SSZ-13. Full size image The simulated catalytic cycles of Zn/SSZ-13 and Cr/SSZ-13 are shown in Supplementary Figs. 34 and 35 , and the calculated energy profiles of ICEC over Zn 3 Cr 1 /SSZ-13, Zn/SSZ-13, and Cr/SSZ-13 are presented in Fig. 4b . The rate-determining step of ICEC is the homolytic cleavage of the β-C-H bond in ethane activation [TS2] (Fig. 4b , Supplementary Table 9 ). Zn 3 Cr 1 /SSZ-13 exhibited a lower activation barrier (2.11 eV) than Zn/SSZ-13 (2.37 eV) and Cr/SSZ-13 (2.23 eV). Moreover, Zn 3 Cr 1 /SSZ-13 also displayed a much lower energy barrier (1.12 eV, 0.73 eV) for CO 2 activation [TS3] and H 2 O formation [TS5] than Zn/SSZ-13 (1.53 eV, 0.94 eV). This explained the much higher CO 2 conversion and utilization of Zn 3 Cr 1 /SSZ-13 catalyst than Zn/SSZ-13 catalyst (Fig. 2b ). We also found that Zn 3 Cr 1 /SSZ-13 exhibited the most favorable energetics of reactants adsorption and products desorption which also helps accelerate catalytic reactions (Supplementary Table 10 ). Therefore, the kinetically and thermodynamically favorable elementary steps in the ICEC catalytic cycle result in the highest catalytic performance of Zn 3 Cr 1 /SSZ-13. Its superior performance in ICEC is due to the atomic synergies between the acidic Zn site and the redox Cr site of ABC. In this study, we demonstrated the advantages of an atomically-synergistic binuclear-site catalyst (ABC) synthesized by colocalizing Zn and Cr sites on a zeolite SSZ-13 support (ZnCr/SSZ-13) for the iso-stoichiometric co-conversion of ethane and CO 2 (ICEC) reaction. This ZnCr ABC catalyst exhibited exceptional catalytic performance, with 100% ethylene selectivity and 99.0% \({{{{{\rm{U}}}}}}_{{{{{{\rm{CO}}}}}}_{2}}\) under optimized conditions. The combined results of XAS, AP-XPS, and DFT studies show that the electronic properties and catalytic activity of ZnCr/SSZ-13 can be precisely assigned to unique atomic synergies between neighboring Zn and Cr atoms resulting from colocalization. The redox Cr site facilitates the formation of Zn δ + , which is the active site for easier adsorption and activation of both ethane and CO 2 . Furthermore, the Cr site accelerates CO 2 dissociation, due to its redox properties, and facilitates the formation and desorption of H 2 O. This combination thus results in rate matching between ethane dehydrogenation and CO 2 hydrogenation. Our study highlights the importance of atomic synergy, providing guidance for developing novel catalysts with potential economic and ecological benefits in CO 2 conversion and olefin production. Materials synthesis. Zn x Cr y /SSZ-13 ( x = 1, y = 0; x/y = 1/2, 1, 2, 3, and 4; x = 0, y = 1) catalysts were prepared by the dry-deposition method [62] . The total amount of Zn and Cr in all catalysts was set at 0.8 mmol per 1 g of support materials. In a typical synthesis, the SSZ-13 zeolite support was pretreated in a vacuum at 120 °C for 3 h to remove moisture. The stoichiometric amount of Zinc (II) acetate and/or chromium (III) acetate hydroxide (Zn + Cr = 0.8 mmol) was thoroughly mixed with 1 g of SSZ-13 zeolites using an analog vortex mixer. The resulting solid mixtures were sufficiently ground in glove box for 20 min. Subsequently, the samples are heated in flowing N 2 (100 mL/min) at 550 °C for 3 h at a ramping rate of 2 °C/min and subsequently in flowing air (100 mL/min) for another 3 h. Both N 2 and air were purified by moisture trap (Restek). Afterward, the resulting materials were pretreated through Na + -neutralization. Typically, the sample was firstly dispersed in deionized water and then dropwise addition of sodium bicarbonate solution (0.01 M, pH = 8) was performed until the solution reached a pH of 7. The slurry was then collected and dried at 110 °C overnight. The samples were finally calcined in static air at 500 °C for 2 h with a ramping rate of 2 °C/min. The final products were stored in an N 2 box. The control samples of Zn x Cr/SSZ-13 (x = 1/2, 1, and 3) were synthesized using the traditional co-precipitation (CP) method according to the reported recipe [41] , followed by Na + neutralization. Materials characterization. Nitrogen physisorption was performed on the Quantachrome Autosorb iQ2 instrument at 77 K to obtain textural information. The surface area (S BET ) was determined from the N 2 isotherms using the Brunauer-Emmett-Teller (BET) method. X-ray fluorescence (XRF) measurements were performed with a EDAX Orbis Micro-XRF Spectrometer. The attenuated total reflection Fourier transform infrared (ATR-FTIR) measurements were conducted by a Thermo Nicolet iS50 FTIR spectrometer with a diamond crystal ATR module. Powder X-ray diffraction (XRD) analysis was performed on a Rigaku MiniFlex 6 G X-Ray Diffractometer (Cu K α radiation with wavelength of 1.5406 Å). The transmission electron microscopy (TEM) experiments were performed on a FEI ThemIS aberration-corrected TEM at the National Center for Electron Microscopy (NCEM) of the Molecular Foundry (MF), Lawrence Berkeley National Laboratory (LBNL). The microscope was operated at 300 keV with a Super-X energy dispersive X-ray spectroscopy (EDS) detector, allowing for rapid chemical identification. X-ray photoelectron spectroscopy (XPS) measurement was conducted at a K-Alpha Plus XPS spectrometer (Thermo Scientific), which consists of a monochromatic Al X-ray source (Al K α = 1,486.68 eV) with variable spot size ranging from 30 microns to 400 microns. Powder samples were placed on a double-sided silver tape and the spectra were acquired using the flood-gun source to account for surface charging. All the spectra were analyzed using the CasaXPS software package. Zn L 3 -edge soft X-ray absorption spectroscopy (sXAS) measurement was performed at Beamline 7.3.1 of the Advanced Light Source (ALS) at Lawrence Berkeley National Laboratory (LBNL). sXAS measurement was collected at room temperature through total electron yield (TEY) mode with a probe depth of no more than 10 nm. All the TEY spectra were normalized to the beam flux. The measurements of Zn K -edge and Cr K -edge XAS spectra including X-ray absorption near edge structure (XANES) and extended X-ray absorption fine structure (EXAFS) were performed at TPS 44 A beamline in National Synchrotron Radiation Research Center (NSRRC) in Taiwan. The data were collected in fluorescence mode by using 7-element silicon drift detector and the Zn and Cr metal foil were used as references for the energy calibration. The data were processed according to standard procedures using Demeter program package. Ambient-pressure XPS (AP-XPS) analysis was conducted at Sandia National Laboratories (Livermore, CA) using a differentially-pumped Al Kα source (Specs model XR50) with a photon energy of 1486.6 keV. Emitted photo- (and Auger) electrons were detected using a near-ambient pressure hemispherical analyzer (Specs model Phoibos 150) mounted in a custom designed system capable of measuring XPS under sample gas pressures up to 10 Torr. We used baked steel gas lines and leak valves to introduce C 2 H 6 (99.995% pure) and CO 2 (99.999% pure) from Matheson Tri-Gas Inc. XPS/Auger peak locations, widths, and areas were obtained using a Shirley background subtraction and by fitting the data to mixed Gaussian-Lorentzian line shapes using CasaXPS software. Performance Tests. The catalytic performance of iso-stoichiometric co-conversion of ethane and CO 2 (ICEC) was conducted on a continuous fix-bed reactor in the temperature range of 400–550 °C and under ambient pressure, which is held inside an electric furnace with temperature controlled by a K-type thermocouple. In a typical catalytic measurement, a total of 200 mg catalyst diluted by 800 mg sand was loaded into the middle of the reactor plugged by quartz wool on two sides. Before the catalytic test, the catalyst bed was pretreated under a flow of Argon (25 sccm) at 550 °C for 1 h with a ramping rate of 10  °C from room temperature. Afterward, the reactant mixtures consisting of 5% CO 2 , and 5% C 2 H 6 balanced with Argon were introduced with a total flow rate of 25 sccm. Argon is used as an internal standard. The reaction products were analyzed by online GC (Agilent 5890, ShinCarbon ST Packed Columns) equipped with thermal conductivity detector (TCD) and flame ionization detector (FID). To better reveal the reaction kinetics, apparent activation barriers were determined in the temperature range of 400–475 °C (The conversions of CO 2 and C 2 H 6 are less than 10%). The carbon and oxygen balances were within 100 ± 2% for all tests. The conversions of CO 2 and C 2 H 6 , C 2 H 4 selectivity, utilization of converted CO 2 ( \({{{{{\rm{U}}}}}}_{{{{{{\rm{CO}}}}}}_{2}}\) ), C 2 H 4 yield, the turnover frequency (TOF) of C 2 H 4 formation, and the space time yield (STY) of C 2 H 4 formation were calculated as follows (where n denotes molar flow of substance (mol/min), n Zn+Cr means the total molar loading of Zn and/or Cr, \({{{{{\rm{M}}}}}}_{{{{{{\rm{C}}}}}}_{2}{{{{{\rm{H}}}}}}_{4}}\) is the molecular weight of C 2 H 4 (28 g/mol) and m cat stands for catalyst mass (kg)): 
    CO_2 conversion  (%)=n_CO_2input-n_CO_2output/n_CO_2input× 100%
 (1) 
    C_2H_6 conversion  (%)=n_C_2H_6input-n_C_2H_6output/n_C_2H_6input× 100%
 (2) 
    C_2H_4 selectivity  (%)=n_C_2H_4output/n_C_2H_6input-n_C_2H_6output× 100%
 (3) 
    U_CO_2(%)=CO_2 conversion/C_2H_6 conversion× 100%
 (4) 
    C_2H_4 yield  (%)=C_2H_6 conversion×C_2H_4 selectivity
 (5) 
    TOF=n_C_2H_4output× 60/n_Zn+Cr
 (6) 
    STY=n_C_2H_4output×M_C_2H_4× 60/1000×m_cat
 (7) It is noted that calculations of \({{{{{\rm{U}}}}}}_{{{{{{\rm{CO}}}}}}_{2}}\) were also calibrated and examined by the equation: 
    U_CO_2(%)=n_CO output/n_C_2H_6input-n_C_2H_6output× 100%
 (8) Computational Methods. All DFT calculations were performed using Vienna ab initio simulation package (VASP) [63] , [64] . The projector-augmented wave (PAW) method was used to represent the core-valence electron interaction [65] , [66] . The generalized gradient approximation (GGA) with the Perdew–Burke–Ernzerhof (PBE) exchange-correlation functional was used with D3 dispersion correction [67] , [68] . The cutoff energy for the planewave basis was 500 eV. To accurately treat the highly localized transition metal 3 d orbitals, the spin-polarized DFT + U approach [69] , [70] was employed: U eff = 4.7 and 3.0 eV were applied to the Zn 3 d and Cr 3 d state, respectively [71] , [72] . Electronic energies were converged to within 10 −4 eV and the atomic positions were relaxed until the force on each atom was less than 0.05 eV/Å. The climbing-image nudged elastic band (CI-NEB) method [73] was used to search for the transition states. A hexagonal unit cell of the SSZ-13 molecular sieve [74] was used as the support: a = b = 13.72 Å, c = 14.95 Å; composition: Na 1 Al 1 Si 35 O 72 . Only the Γ-point was used to sample the Brillouin zone. The unit cell contains two hexagonal prisms; two units of Zn 2 O 2 and Cr 2 O 3 were placed on the two prisms, to create the models of Zn/SSZ-13 and Cr/SSZ-13, respectively; one Zn 2 O 2 unit was placed on one of the prisms and one ZnCrO 2 unit on the other, to create the model of Zn 3 Cr 1 /SSZ-13 (see Supplementary Fig. 30 ).